Strain-engineered manufacturing of freeform carbon nanotube microstructures The skins of many plants and animals have intricate microscale surface features that give rise to properties such as directed water repellency and adhesion, camouflage, and resistance to fouling. However, engineered mimicry of these designs has been restrained by the limited capabilities of top–down fabrication processes. Here we demonstrate a new technique for scalable manufacturing of freeform microstructures via strain-engineered growth of aligned carbon nanotubes (CNTs). Offset patterning of the CNT growth catalyst is used to locally modulate the CNT growth rate. This causes the CNTs to collectively bend during growth, with exceptional uniformity over large areas. The final shape of the curved CNT microstructures can be designed via finite element modeling, and compound catalyst shapes produce microstructures with multidirectional curvature and unusual self-organized patterns. Conformal coating of the CNTs enables tuning of the mechanical properties independently from the microstructure geometry, representing a versatile principle for design and manufacturing of complex microstructured surfaces. Scalable fabrication of microstructures that mimic the hierarchical surface designs found in nature has been a long-standing aspiration of material scientists [1] , [2] , [3] , [4] , [5] . While symbiotic growth of the integrated circuit and microelectromechanical systems (MEMS) industries has enabled innovations in three-dimensional (3D) fabrication that leverage semiconductor processing tools, these methods, such as interference or inclined exposure lithography, are typically limited to arrays of identical structures [6] , [7] , [8] . Rapid prototyping methods such as direct laser writing, multiphoton lithography and focused ion beam milling can create arbitrary forms but are serial, and therefore have lower areal throughput [9] , [10] . It is also especially difficult to fabricate surface structures having curved and/or re-entrant geometries. On the other hand, use of locally directed actions, such as mechanical stresses, capillary forces and electromagnetic fields, along with their interactions with templates, offers opportunity to create novel self-organized geometries and to design fabrication processes that achieve attractive combinations of dimensional control and throughput [2] , [8] , [11] , [12] , [13] , [14] , [15] . Examples abound in soft materials and chemical systems including microscale reaction-diffusion patterns [16] , [17] , self-assembly of block copolymers [18] and helical aggregation of polymer nanopillars [19] , [20] . However, many of these processes need further development to achieve high production rates and uniformity over large areas. We present a novel approach taking advantage of microscale top–down lithographic patterning in conjunction with nanoscale self-organization, which enables large-area fabrication of freeform microstructures made of aligned carbon nanotubes (CNTs). This process leverages the influence of the catalyst–substrate interactions on the growth rate of CNTs [21] , creating strain gradients during synthesis that guide the CNTs into curved microscale geometries. Our method is analogous to the well-known use of thin-film stress to create curved and folded MEMS structures [22] . However, because our process is based on an additive chemical synthesis process instead of a subtractive etching and release technique, it enables the direct synthesis of complex microstructures that are perpendicular rather than parallel to the substrate. This has two major implications: it enables fabrication of closely packed arrays of structures with heterogeneous shapes, and the porosity of the CNT forests enables conformal coating after growth to modify chemical and/or mechanical properties. We demonstrate this latter point by conformal coating of CNT ‘microtruss’ arrays by atomic layer deposition (ALD) and polymer chemical vapour deposition (CVD), which increases their mechanical stiffness without changing the geometry. Fabrication CNTs grown by CVD from a high-density arrangement of catalyst nanoparticles on a substrate are known to self-organize into vertically aligned assemblies often called ‘CNT forests’ [23] , [24] . We first observed that the density and rate of CNT forest growth from a supported catalyst (Fe/Al 2 O 3 , 1/10 nm) can be influenced by the material immediately beneath the support. This premise is shown in Fig. 1a ; patterning of CNT growth catalyst (Fe/Al 2 O 3 ) on a SiO 2 /TiN ‘checkerboard’ followed by exposure to standard CVD conditions (see Methods) results in a bi-level CNT micropillar array. The catalyst patterns directly on SiO 2 grow CNTs to ~100 μm (in <2 min), whereas the patterns on TiN (on SiO 2 ) grow CNTs to 50 μm in the same time span. In Fig. 1b , tri-level CNT forests are grown by arranging patches of catalyst on SiO 2 , 70 nm TiN and 140 nm TiN. This principle could be extended to an arbitrary number of levels or even continuous height gradients via additional lithography and underlayer deposition steps that modulate the growth rate via catalyst–substrate interactions. 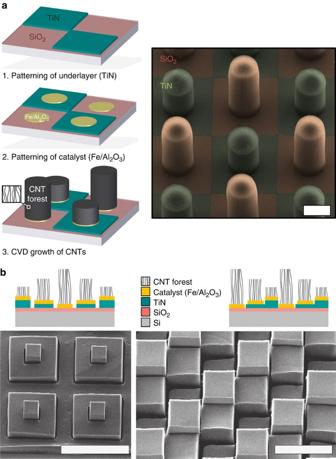Figure 1: Multi-height CNT micropillar growth using TiN as a rate-controlling catalyst underlayer. (a) Process steps including two lithography steps, and accompanying (colour added) pattern of cylindrical CNT micropillars grown on ‘checkerboard’ of alternating TiN (80 nm thickness) squares on SiO2. Scale bar, 40 μm. (b) Tri-level arrays made by substrate and catalyst patterning with three lithography steps (TiN layers are 40 nm and 80 nm thickness). Scale bar, 500 μm (left) and 200 μm (right). Figure 1: Multi-height CNT micropillar growth using TiN as a rate-controlling catalyst underlayer. ( a ) Process steps including two lithography steps, and accompanying (colour added) pattern of cylindrical CNT micropillars grown on ‘checkerboard’ of alternating TiN (80 nm thickness) squares on SiO 2 . Scale bar, 40 μm. ( b ) Tri-level arrays made by substrate and catalyst patterning with three lithography steps (TiN layers are 40 nm and 80 nm thickness). Scale bar, 500 μm (left) and 200 μm (right). Full size image Next we used the above differential growth principle to design compound catalyst/underlayer patterns that directly form curved CNT forest geometries. If a continuous microscale catalyst pattern is placed partially on SiO 2 and partially on TiN, the differential growth rates induce stress within the CNT microstructure. For example, as shown in Fig. 2a,b , a square catalyst pattern with half of its area on the TiN layer bends towards the side which is on TiN, due to the difference in growth rate on the coupled halves of the structure. The stress is transferred between contacting CNTs at the boundary region via mechanical entanglement and van der Waals interactions among the CNTs. Depending on the curvature and length of the structures, slanted micropillars ( Fig. 2a ) or arches ( Fig. 2b ) can be fabricated. Because the local interaction and differential growth rate determine the trajectory of each structure, large arrays with nearly identical anisotropic shapes can be produced as shown in the scanning electron microscopy (SEM) images. Importantly, substrate preparation for growth of these 3D structures requires only two standard photolithography steps, one for patterning the TiN layer and one for patterning the catalyst layer. 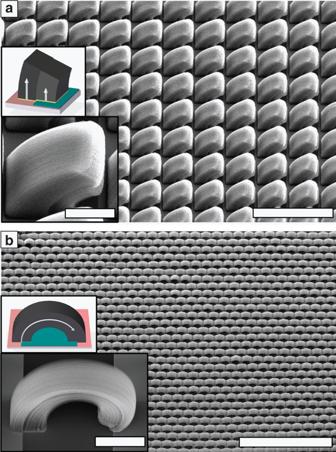Figure 2: Curved CNT micropillars. The micropillars are grown from catalyst rectangles partially overlapping TiN (shown as green layer in the schematics, see inset) and bend towards the TiN side, which grows more slowly and couples to the faster-growing region of catalyst directly on SiO2. (a) Closely spaced short structures with ~45° takeoff angle. Scale bar, 100 μm (panel) and 20 μm (inset). (b) Arch-like structures that curve over and contact the substrate at their distal ends. Scale bar, 200 μm (panel) and 20 μm (inset). Figure 2: Curved CNT micropillars. The micropillars are grown from catalyst rectangles partially overlapping TiN (shown as green layer in the schematics, see inset) and bend towards the TiN side, which grows more slowly and couples to the faster-growing region of catalyst directly on SiO 2 . ( a ) Closely spaced short structures with ~45° takeoff angle. Scale bar, 100 μm (panel) and 20 μm (inset). ( b ) Arch-like structures that curve over and contact the substrate at their distal ends. Scale bar, 200 μm (panel) and 20 μm (inset). Full size image The curvature can be controlled by designing the amount of overlap between the catalyst and the TiN underlayer. This is illustrated in Fig. 3a,b , which respectively shows arrays of round and square cross-section micropillars where the overlap distance is varied from left to right (increments of 5 μm). As expected, the portion of the pillars growing on TiN is always shorter, and as a result, all pillars bend towards the TiN side. As the portion of overlap decreases, the stress induced by the differential growth rate causes increased bending (smaller radius of curvature), reaching a maximum when the catalyst shape is split symmetrically by the TiN layer. With <50% overlap on TiN, the curvature increases gradually until the structure is only slightly curved at the rightmost extent of the array. The CNTs are generally tangential to the curvature of the microstructures, owing to the intrinsic CNT alignment observed in vertical CNT forests. 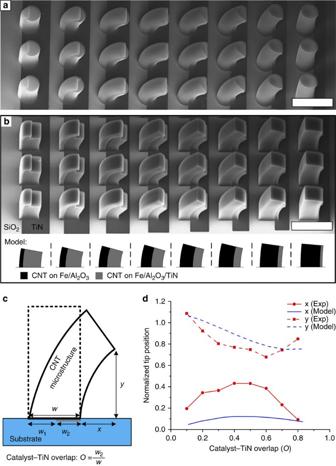Figure 3: Shape gradients and their use in elementary modelling of the stress-driven CNT growth process. (a,b) Arrays of round and square CNT micropillars with decreasing catalyst/TiN overlap from left to right. Scale bar, 100 μm. (c) Schematic of geometric parameters used to quantify deformation of square micropillars. (d) Output of differential expansion model predicting vertical and lateral deflection versus substrate pattern design, comparing simulations (inset tob), and measurements from SEM images. Figure 3: Shape gradients and their use in elementary modelling of the stress-driven CNT growth process. ( a , b ) Arrays of round and square CNT micropillars with decreasing catalyst/TiN overlap from left to right. Scale bar, 100 μm. ( c ) Schematic of geometric parameters used to quantify deformation of square micropillars. ( d ) Output of differential expansion model predicting vertical and lateral deflection versus substrate pattern design, comparing simulations (inset to b ), and measurements from SEM images. Full size image Static model of stress-driven CNT curvature The coupling of stress and CNT growth rate, via the anisotropic mechanics of the CNT forest [25] , is a complex problem. However, we find that a static mechanical model analogous to that used for differential expansion of a bi-material cantilever beam can reasonably predict the curvature of CNT structures grown from an overlapped catalyst/TiN rectangle. Starting from the classical formulation of the bimetallic strip model [26] , we replace the temperature-dependent expansion term by a differential lengthening term representing the CNT growth rate. Accordingly, the curvature of the compound CNT microstructure is described as: Here ρ is the radius of curvature, R 1 and R 2 are the growth rates (1 denotes CNTs on Fe/Al 2 O 3 /SiO 2 and 2 denotes CNTs on Fe//Al 2 O 3 /TiN) and w is the CNT micropillar width. In addition, m and n are defined as where w denotes the width and E denotes the respective Young’s Moduli of the segments. The value of n is specified as 0.6, which is the ratio of the measured areal mass density of CNTs on the respective underlayers; however, because the elongation of each layer is specified in the model, the output is insensitive to this value. The geometric parameters are defined in Fig. 3c . Using the calculated curvatures and the weighted average growth rate, the shapes of the resultant CNT microstructures were visualized using Matlab. The simulation results correspond to the rows of structures in the SEM image Fig. 3b . To compare the experiments with the simulation, the tip position was characterized in horizontal and vertical axes, normalized to the base dimension ( w ), as shown in Fig. 3c . For both the experiment and simulation, the x position of the tip reaches its maximum at 0.4 overlap, and the y position reaches its minimum at ~0.6–0.7 overlap. The differences between the simulated and calculated displacements arise because the model does not capture the exact kinetics of CNT growth, which varies with time. Moreover, it cannot consider how the stress between the two portions of the structure, which are idealized as perfectly coupled without slip, influences the deformation. CNT forests have anisotropic mechanical properties, with the lateral stiffness (perpendicular to the CNT alignment) typically much less than the axial stiffness [25] , therefore, in principle, favouring greater deflection due to the built-in stress gradient. To gain further insight into the mechanical coupling causing stress-driven bending, we designed a ‘striped’ structure where alternate catalyst/underlayer regions are coupled with a large interfacial area. This structure is symmetric, so it grows straight vertically yet has significant internal stresses. As shown in Fig. 4a and the neighbouring insets, the faster-growing CNTs deform collectively into a wavelike pattern. Therefore, while the vertical growth rate of the structure is matched at the interface, the faster-growing side still accumulates longer CNTs and these CNTs bend and possibly buckle to accommodate their additional length. This deformation mode is similar to what is observed in mechanically compressed CNT forests [27] . Local wrinkling and buckling of the CNTs in the compound microstructures ( Fig. 4a ) indicates that the growth stress causes complex mechanical deformations, which cannot be predicted by linear elasticity and the bimaterial deflection model. 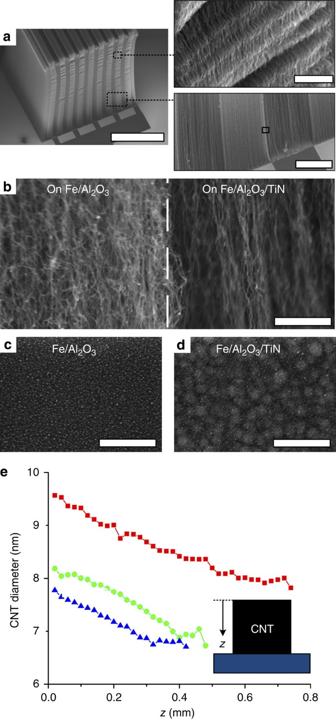Figure 4: Analysis of CNT morphology. (a) SEM image of micropillar with catalyst on fine stripes of TiN, with close-up images showing the CNT morphology difference and evidence of internal stress causing local deformation. Scale bar, 100 μm (left), 2 μm (upper right) and 10 μm (lower right). (b) Close-up images of the aligned CNT morphology in adjacent segments of the micropillar. Scale bar, 500 nm. (c,d) SEM images of the substrate morphology after annealing in H2 and rapid cooling, showing hierarchical morphology of nanoparticles on the catalyst/TiN area. Scale bar, 500 nm. (e) Diameter mapping within the CNT forests, from fitting of SAXS data. Red—CNT of Fe/Al2O3, Green—CNT on Fe/Al2O3/TiN (40 nm), and Blue—CNT on Fe/Al2O3/TiN (80 nm). Figure 4: Analysis of CNT morphology. ( a ) SEM image of micropillar with catalyst on fine stripes of TiN, with close-up images showing the CNT morphology difference and evidence of internal stress causing local deformation. Scale bar, 100 μm (left), 2 μm (upper right) and 10 μm (lower right). ( b ) Close-up images of the aligned CNT morphology in adjacent segments of the micropillar. Scale bar, 500 nm. ( c , d ) SEM images of the substrate morphology after annealing in H2 and rapid cooling, showing hierarchical morphology of nanoparticles on the catalyst/TiN area. Scale bar, 500 nm. ( e ) Diameter mapping within the CNT forests, from fitting of SAXS data. Red—CNT of Fe/Al 2 O 3 , Green—CNT on Fe/Al 2 O 3 /TiN (40 nm), and Blue—CNT on Fe/Al 2 O 3 /TiN (80 nm). Full size image As seen in Fig. 3a and supplementary Fig. 1a , some structures separate at the interface between the differentially growing regions, due to shear stresses at the interface. In future work, this could be remedied by adapting the structure design to reduce the interfacial shear stress between the segments, or by using a more gradual growth rate gradient to accommodate the stress gradient, such as a three-layer design as in Fig. 1b . However, we importantly find that structures that do not separate during synthesis can withstand large subsequent deformations without failure. For instance, Supplementary Fig. 1b shows an SEM image of an arrangement of bent pillars during compression to 50% vertical strain, at which point delamination at the interface begins only where the pillars kink near their midsection. CNT and catalyst morphology The strain-engineered CNT microstructures show differing CNT density and alignment in the fast- and slow-growing portions. In Fig. 4a,b , the CNTs grown from catalyst on TiN appear to have greater vertical alignment influenced by the interface with the faster-growing region. On the other hand, the CNTs grown from catalyst on SiO 2 are less aligned, due to the retarding force from the slower-growing mating regions. We hypothesized that the differential CNT growth behaviour on the TiN underlayer may be attributed to differences in the catalyst morphology, which can influence the CNT diameter distribution and number density. Atomic force microscopy showed that the as-deposited catalyst layers on SiO 2 and TiN have a similar topology ( Supplementary Fig. 2 ). However, on annealing in H 2 /He before hydrocarbon exposure (see Methods), the TiN–catalyst layer forms shallow mounds, tens of nanometres high and hundreds of nanometres wide, in addition to smaller catalyst particles. The control case of catalyst on SiO 2 does not exhibit such topography. For samples with 80 nm TiN layer, the average catalyst particle height and spacing were calculated to be 5.2 and 19 nm, respectively. Compared with those on SiO 2 (7.5 and 18 nm, respectively [28] ), the catalyst particle sizes are smaller on average while the spacing is comparable. In addition, the root mean square roughness of the annealed catalyst/TiN layer is 5.6 nm, which is considerably higher than that of catalyst on SiO 2 (1.4 nm). Small angle X-ray scattering (SAXS) was used to further investigate the CNT forest morphology [29] , [30] . For this experiment, CNTs were grown for 10 min on SiO 2 and on 40 and 80 nm TiN layers; these samples reached lengths of 800, 500 and 400 μm, respectively. The scattered X-ray intensities were fitted to a mathematical form factor model for hollow cylinders [31] to calculate the diameter and the Herman’s orientation parameter, which is a measure of alignment. Both the CNT diameter ( Fig. 4e ) and alignment ( Supplementary Fig. 3 ) are shown to be lesser for increasing TiN underlayer thickness. Specifically, CNTs on SiO 2 have initial average diameter of approximately 8.5 nm, while CNTs on TiN are approximately 7.5 nm in diameter. These measurements further support the atomic force microscopy data, which showed that the catalyst particles on TiN layers are smaller than those on SiO 2 . The decrease in diameter with growth time has been attributed to diffusion of the catalyst into the Al 2 O 3 (refs 29 , 32 ). The Herman’s orientation parameter increases from the top of the forest (the initial growth), reaches a maximum and then decreases towards the bottom of the forest. This trend is typically observed for CNT forests grown by CVD, and has been attributed to density variation due to collective activation and deactivation of the growing CNT population [29] . The measured areal mass density of the CNT forests is 0.011 mg mm −2 on 80 nm TiN and 0.018 mg mm −2 on SiO 2 . Although we have not directly compared the mechanical properties of the different segments, we expect that the CNT forests on TiN have lower stiffness and lesser anisotropy in mechanical properties. The positive correlation between CNT density and alignment is also expected based on recent literature, which demonstrated that CNT-CNT crowding controls alignment within non-patterned forests [33] . On the basis of our understanding of the elementary catalyst/underlayer designs that achieve unidirectional bending, we designed a variety of more complex patterns that produce exemplary CNT microstructures having complex curvature. For instance, a compound shape consisting of a ‘+’ catalyst microfeature with each arm offset by a rectangular TiN underlayer results in growth of twisted CNT microstructures ( Fig. 5a ), resembling macroscale propellers. The first-order applicability of the bimaterial bending model discussed above inspired us to evaluate the suitability of finite element modeling to predict the shapes of these structures. These were simulated using COMSOL finite element modeling software as illustrated in Fig. 5a , capturing the uncoupled differential growth rate ( Fig. 1a ) as a 50% expansion mismatch and estimating the Young’s modulus as 30 MPa for the CNTs on TiN and 50 MPa on SiO 2 (ref. 34 ). 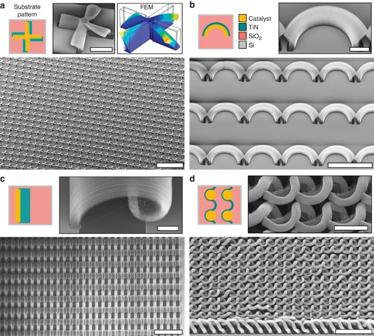Figure 5: Design and fabrication of arrays of complex microstructures. Each of the four panels contains a sketch (top left) of the catalyst–TiN pattern used for CNT growth, a close-up SEM image (top right) and an exemplary array of structures (bottom). (a) Twisted propeller-like structures, made from azimuthally offset crosshair catalyst/TiN layers, also compared with finite element model (FEM) prediction of shape (top right). Scale bar, 40 μm (top right) and 500 μm (bottom). (b) Outward curving semicircles made from radially offset catalyst/TiN layers. Scale bar, 5 μm (top right) and 100 μm (bottom). (c) Scroll-like deformation of thin-walled microstructures with slight catalyst/TiN overlap. Scale bar, 10 μm (top right) and 250 μm (bottom). (d) Collective organization of bending microstructures into a wavy pattern. Scale bar, 10 μm (top right) and 40 μm (bottom). Figure 5: Design and fabrication of arrays of complex microstructures. Each of the four panels contains a sketch (top left) of the catalyst–TiN pattern used for CNT growth, a close-up SEM image (top right) and an exemplary array of structures (bottom). ( a ) Twisted propeller-like structures, made from azimuthally offset crosshair catalyst/TiN layers, also compared with finite element model (FEM) prediction of shape (top right). Scale bar, 40 μm (top right) and 500 μm (bottom). ( b ) Outward curving semicircles made from radially offset catalyst/TiN layers. Scale bar, 5 μm (top right) and 100 μm (bottom). ( c ) Scroll-like deformation of thin-walled microstructures with slight catalyst/TiN overlap. Scale bar, 10 μm (top right) and 250 μm (bottom). ( d ) Collective organization of bending microstructures into a wavy pattern. Scale bar, 10 μm (top right) and 40 μm (bottom). Full size image Similarly, thin semicircles of CNTs can be directed to curve outward by offsetting the TiN underlayer as shown in Fig. 5b . Further structural complexity is shown by the scrolling of thin offset rectangular patterns ( Fig. 5c ). Finally, exotic hierarchical arrangements can be formed by the interaction of closely spaced structures, such as the self-organization of offset circular micropillars into wavy patterns ( Fig. 5d ) that are reminiscent of macroscale crochet stitching. We hypothesize that, after the individual structures bend unidirectionally and contact one another, their continued growth and steric hindrance cause the wavy pattern to form. More investigation is needed to understand the complex deformations of these structures, and their relationship to the mechanics of the CNT forest and the mechanical feedback on the growth process itself. Notably, in spite of the complex geometries and local deformations, all of these structures can be produced with impressive consistency over large arrays. Arrays of several hundred structures were examined and shown to exhibit nearly identical forms, with defects most frequently arising from debris due to the lithography process rather than the CNT growth step. In this study, we explored structures with critical dimensions as small as 5 μm ( Fig. 5 ) and found that the uniformity of the structures was not sacrificed at this scale. We expect that smaller 3D microstructures could be made while still using optical lithography along with high-precision alignment of the catalyst and TiN layers. Notably, others have fabricated sub-micron vertical CNT features for use as interconnects [35] . Further, because the curved and twisted geometries result from collective behaviour of CNT forest growth, we expect the structures to require a certain minimal size to average out the stochastic variation of individual CNT growth rate and catalyst lifetime. Considering the approximate CNT-CNT spacing within the current microstructures (~100 nm), the minimal feature size of reliable growth of curved microstructures may be limited to ~1 μm, although this requires further investigation. Finally, we show that 3D CNT structures can be post-processed via both wet and dry methods that enable tuning of their properties and functionality. Low-density bent CNT micropillars can be transformed into robust, densely packed CNT structures by capillary forming ( Fig. 6a,b ) [34] , [36] , [37] . To do so, the substrate is exposed to a stream of heated acetone vapour, causing acetone to condense onto the CNTs and substrate, and infiltrate each CNT microstructure. On subsequent evaporation of the acetone, the CNT forest shrinks laterally, due to the surface tension of the shrinking meniscus. Previously, we showed that capillary forming of vertical CNT microstructures increases the Young’s modulus in compression ~100-fold, from ~50 MPa to 4 GPa [34] . These values are comparable to soft rubbers and stiff epoxies, respectively. Moreover, in the present case, the capillary forming process preserves the curved geometry and increases the lateral deflection of the micropillars. 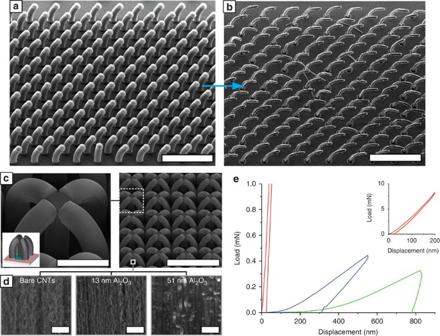Figure 6: Post-processing of 3D CNT microstructures. (a,b) Array of bending micropillars before and after capillary forming, respectively. The unidirectional anisotropic morphology is maintained and the micropillar cross-section decreases, while the lateral deflection angle of the structures increases. Scale bar, 200 μm. (c) Microtruss array fabricated to study mechanical reinforcement by vapour phase coating of the CNTs. Scale bar, 100 μm (left) and 400 μm (right). (d) SEM images of aligned CNTs in the forest sidewall before and after coating with Al2O3by atomic layer deposition (ALD). Scale bar, 1 μm. (e) Load-displacement curves before and after ALD coating, where the stiffness is measured from the slope of the unloading curve. Green—no coating, blue—Al2O3coating (ALD, 100 cycles), and red—Al2O3coating (ALD, 1,000 cycles). Figure 6: Post-processing of 3D CNT microstructures. ( a , b ) Array of bending micropillars before and after capillary forming, respectively. The unidirectional anisotropic morphology is maintained and the micropillar cross-section decreases, while the lateral deflection angle of the structures increases. Scale bar, 200 μm. ( c ) Microtruss array fabricated to study mechanical reinforcement by vapour phase coating of the CNTs. Scale bar, 100 μm (left) and 400 μm (right). ( d ) SEM images of aligned CNTs in the forest sidewall before and after coating with Al 2 O 3 by atomic layer deposition (ALD). Scale bar, 1 μm. ( e ) Load-displacement curves before and after ALD coating, where the stiffness is measured from the slope of the unloading curve. Green—no coating, blue—Al 2 O 3 coating (ALD, 100 cycles), and red—Al 2 O 3 coating (ALD, 1,000 cycles). Full size image Alternatively, curved CNT microstructures can be coated conformally via vapour phase methods, thereby enabling decoupled control of geometry and mechanical properties. To investigate this, we fabricated CNT ‘microtruss arrays’ ( Fig. 6c–e ), which are analogous to truss designs used in composite materials to achieve high strength and energy absorption at relatively low density [38] , [39] , [40] . The CNT microtrusses each consist of four corner members and a central pillar, meeting at an apex. We explored coating of the CNT microtrusses with both parylene (by CVD; Supplementary Fig. 4 ) and alumina (by atomic layer deposition; Fig. 6d ). On vapour phase infiltration of the precursors, the CNTs and bundles within the forest are coated individually and conformally [41] , enabling fine-tuning of their porosity and mechanics without altering the microstructure geometry. Via flat punch compression testing, we found that a 51 nm Al 2 O 3 coating on the CNTs increases the mechanical stiffness by more than 100-fold; typical loading–unloading curves are shown in Fig. 6e and Supplementary Fig. 4 for different coating materials and thicknesses. The equivalent stiffness range of the 3D CNT microtrusses is 0.36–54 kN m −1 , which spans typical values of MEMS springs used in probe card arrays [42] . A further attribute of the TiN underlayer is its electrical conductivity. In the future, electrical integration of strain-engineered CNT structures in conjunction with the post-processing methods described above could be useful in advanced microsystems, including as structural elements or microsensors [43] , [44] . Such applications could take advantage of the thermal and mechanical durability of CNTs, as well as the anisotropic properties arising from their alignment and collective curvature. The ability to fabricate large arrays of 3D microstructures is also conducive to mimicry of nature’s advanced functional materials [5] . We say this because the structures shown in Figs 2 and 5 have similar size and geometry to features on butterfly wings that have anisotropic wetting properties [45] , dry adhesive contacts on the legs of beetles and gecko lizards [3] , and microscale sensing hairs found on spiders [46] . Therefore, we suggest that 3D CNT microstructures offer opportunities to further engineer the excellent dry adhesive [47] , [48] and superhydrophobic [49] properties previously reported for CNT forests. For mechanical applications such as dry adhesion, an important consideration is the adhesion of the structures to the substrate, as well as the mechanical resilience of the structures on repeated loading. While we have found that the segments of the curved structures are well adhered to each other ( Supplementary Fig. 1b ), we anticipate that coating or transfer steps may be necessary to anchor the structures for use as robust surface contacts [48] . Exploration of potential optical and photonic applications would require further miniaturization of the structures. Nevertheless, combined with the emerging methods to grow and pattern CNT forests on large-area substrates [50] , [51] , [52] , we are optimistic that the methods shown here can enable large-area surface coatings having advanced functionalities. In summary, we show that strain-engineered CNT growth enables the scalable fabrication of complex 3D microstructures having unidirectional and multidirectional curvature. The capability to produce such structures en masse using only 2D patterning methods along with standard thermal processing contrasts the limitations of many existing processes that require serial processing or sequential exposure using complex inclined lithography methods. Moreover, the structures can profit from the mechanical robustness and electrical conductivity of CNTs, and their mechanical and surface properties can be engineered independently from their geometry by conformal coating of the CNTs after growth. This represents a highly attractive principle for materials design, and is promising for scalable manufacturing of 3D microstructured surfaces having biomimetic properties. Substrate patterning and CNT growth The catalyst and TiN layers are patterned on (100) silicon wafers coated with 300 nm of thermally grown SiO 2 . Each layer is patterned by lift-off processing, by photolithography (photoresist IX845) followed by ultrasonic agitation in acetone. The TiN layer is deposited and patterned first, and then the catalyst layer (1 nm Fe on 10 nm Al 2 O 3 ) is deposited and patterned. The wafer is then diced into ~1 × 1 cm pieces, the substrates are placed in the quartz tube furnace and the CNT growth is performed. The recipe starts by with flowing 100/400 s.c.c.m. of He/H 2 while heating to 775 °C over 10 min (ramping step); then the system is held at 775 °C for 10 min (annealing step) while maintaining the gas flow. Then 100 s.c.c.m. of C 2 H 4 is added to the gas mixture at 775 °C for CNT growth for the desired duration. The typical growth rate is ~50 μm min −1 on Fe/Al 2 O 3 /SiO 2 . Once the CNTs have grown, C 2 H 4 is removed from the gas mixture and the furnace is cooled to <100 °C. After cooling, the system is purged with He before the sample is removed. Optionally, C 2 H 4 flow can be maintained while cooling down to improve the adhesion of the CNT microstructures to the substrate. Once the cooling step is complete, the quartz tube is purged with 1,000 s.c.c.m. of He for 5 min before opening up the end caps and retrieving the samples. Small angle X-ray scattering SAXS characterization of CNT microstructures was performed at the Cornell High Energy Synchrotron Source using the G1 beamline (10±0.1 keV, 0.13 nm wavelength). The beam is focused to a 10 μm spot using a single bounce monocapillary. The CNT sample is placed on a motorized stage and the focused X-ray beam is passed through the sample. The scattered beam is collected using a 2D detector and the measured intensities normalized to the original intensity measured by another detector at upstream of the CNT sample. The scattering data are then fitted to a mathematical model assuming a log-normal distribution of hollow cylinders to calculate the CNT diameters as well as the Herman’s parameter for CNT alignment. The detailed procedure is described by Bedewy et al. [29] How to cite this article: De Volder, M. et al. Strain-engineered manufacturing of freeform carbon nanotube microstructures. Nat. Commun. 5:4512 doi: 10.1038/ncomms5512 (2014).